Interlayer gap widened α-phase molybdenum trioxide as high-rate anodes for dual-ion-intercalation energy storage devices 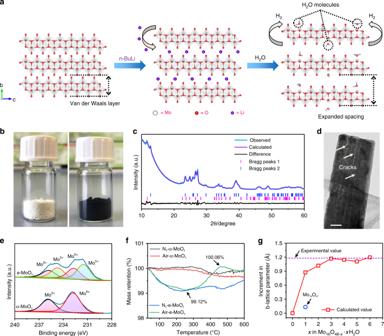Fig. 1: Structure and composition analysis of α-MoO3and e-MoO3. aSchematic representation of expansion process from pristine α-MoO3(left), reaction withn-butyllithium (middle), to e-MoO3with H2O molecules located at the oxygen-defect sites (right). White: Mo; Red: O; Purple: Li; Blue: H.bDigital photos of α-MoO3(left) and e-MoO3(right).cRietveld refinement of XRD pattern anddhigh-resolution TEM image for e-MoO3.Scale bar ind50 nm.eMo 3d XPS profiles of α-MoO3and e-MoO3.fTGA curves of α-MoO3and e-MoO3measured in nitrogen and air atmosphere.gCalculated increment inb-lattice parameter induced by H2O intercalation. The value is also compared with the calculated value of oxygen-defective MoO3−x(Mo16O47) and experimental value. Employing high-rate ion-intercalation electrodes represents a feasible way to mitigate the inherent trade-off between energy density and power density for electrochemical energy storage devices, but efficient approaches to boost the charge-storage kinetics of electrodes are still needed. Here, we demonstrate a water-incorporation strategy to expand the interlayer gap of α-MoO 3 , in which water molecules take the place of lattice oxygen of α-MoO 3 . Accordingly, the modified α-MoO 3 electrode exhibits theoretical-value-close specific capacity (963 C g −1 at 0.1 mV s −1 ), greatly improved rate capability (from 4.4% to 40.2% at 100 mV s −1 ) and boosted cycling stability (from 21 to 71% over 600 cycles). A fast-kinetics dual-ion-intercalation energy storage device is further assembled by combining the modified α-MoO 3 anode with an anion-intercalation graphite cathode, operating well over a wide discharge rate range. Our study sheds light on a promising design strategy of layered materials for high-kinetics charge storage. Triggered by a huge energy demand from various industries ranging from individual electronics to grid storage, electrochemical energy storage devices represent an active field for both research development and practical applications [1] , [2] , [3] , [4] . Typically, supercapacitors and batteries differ in electrochemical mechanisms, hence featuring almost opposite energy and power characteristics [5] , [6] , [7] , [8] . However, the demand for power and energy supply is equally imperative in actual use and is keen to expand in the future. Thus it is highly desirable to design new electrochemical energy storage technologies to mitigate the trade-off between power density and energy density [9] . Recently, the dual-ion energy storage (DIES) concept has attracted increasing attention as it holds different charge storage chemistry with the conventional “rocking-chair” mechanism [10] , [11] , [12] , [13] . In DIES devices, the electrolyte provides both cations and anions to be involved in charge storage. Graphitic carbon provides an ideal host for anion accommodation. The high anion-intercalating potential (>4.0 V vs. Li/Li + ) and ultrafast rate capability (78% capacity retention, up to 100 C rate) enable graphitic carbon a promising cathode for constructing energy storage devices with both high energy and power densities [14] . Previous studies have proposed several new DIES devices by assembling graphite cathode with conventional battery-type anodes (such as Li metal [14] , graphite [15] , Al metal [16] , Sn metal [17] , WS 2 [18] , etc.). However, the power performance of DIES devices is still limited, and there is great interest in designing high-rate pseudocapacitive anode to be combined with graphite cathode to assemble high-energy, high-power DIES device. Orthorhombic MoO 3 (α-MoO 3 ) is composed of edge-sharing [MoO 6 ] octahedra bilayers stacked along [010] by van der Waals (vdW) interaction. It has been considered as one of the most promising cation-intercalation materials due to its eco-friendliness and also high Mo 6+ /Mo 4+ redox activity [19] , [20] . The Li + -intercalation reaction in α-MoO 3 involves both Mo 6+ /Mo 5+ and Mo 5+ /Mo 4+ redox couples, which makes α-MoO 3 a promising electrode for Li-ion storage with a theoretical capacity of 1005 C g −1 [21] . Also, the electrochemical potential for Li-ion intercalation (around 2–3 V vs. Li/Li + ) is far below the anion-intercalation potential of graphitic carbon (>4.0 V vs. Li/Li + ), which suggests the promise for assembling DIES devices composed of MoO 3 anode and graphite cathode. However, the widespread application of α-MoO 3 is severely restricted by its modest electrochemical reaction kinetics due to the low charge/ion transport efficiency, leading to poor rate capability of α-MoO 3 electrodes [19] , [22] . In addition, the unfavorable phase transition of α-MoO 3 electrode around 2.8 V vs. Li/Li + during the initial lithiation process results in the distortion of layers and a rapid capacity decay during the cycling test [23] , [24] . To tackle these obstacles, previous studies employed approaches like constructing nanostructures [25] and creating oxygen vacancy [26] to obtain favorable α-MoO 3 electrode with pseudocapacitive charge storage behavior and acceptable cycling life. Nevertheless, those reported α-MoO 3 electrodes presented unsatisfied areal capacity performance due to low electrode weight loading (e.g., 39 mC cm −2 at 1 mV s −1 with mass loading of 40 μg cm −2 ) [26] . Such low areal performance limits the practical interest of these electrodes in energy storage devices, since it would result in a drastic decrease in performance at the cell level [27] . In this study, we widen the interlayer gaps of α-MoO 3 by incorporating H 2 O molecules between vdW interlayers (α-MoO 3 with expanded interlayer gaps is denoted as e-MoO 3 ). The incorporated H 2 O molecules take the place of lattice O of α-MoO 3 and expand the ionic channel dimension, which is evidenced by the obviously increased b -lattice parameter of e-MoO 3 (15.02 Å) compared to α-MoO 3 (13.85 Å). e-MoO 3 electrode prepared from this approach exhibits a high specific capacity (963 C g −1 or 578 mC cm −2 at 0.1 mV s −1 ), remarkably improved electrochemical reaction kinetics with boosted rate performance (e-MoO 3 vs. α-MoO 3 : 40.2% vs. 4.4% capacity retention at 100 mV s −1 ) as well as cycling life (e-MoO 3 vs. α-MoO 3 : 71% vs. 21% capacity retention over 600 cycles) during Li + storage. Finally, we assemble a DIES device combining a Li + -intercalation e-MoO 3 anode together with a PF 6 − -intercalation graphite cathode in 2 M LiPF 6 electrolyte. Taking advantage of the fast-kinetics intercalation/de-intercalation processes at both anode and cathode, the as-assembled DIES device operates within a 1.0–3.5 V voltage window over a wide discharge rate range (discharge time from 25 s to 3.5 h), and shows high energy density (up to 44 Wh L −1 based on the whole device) with decent power capability (600 W L −1 ). Expanding the interlayer gaps of α-MoO 3 The procedure for expanding interlayer gaps of pristine α-MoO 3 is described in Fig. 1a . α-MoO 3 nanowires were first synthesized through a hydrothermal method and further immersed for 12 h in a solution of n -butyllithium dissolved in hexane. Fast color change from white to dark blue was observed (Fig. 1b ), suggesting the creation of reduced Mo species due to Li + intercalation [19] , [26] . Afterwards, the sample was transferred into water, resulting in the oxidation of the sample by Li + removal and simultaneous reduction of water into gaseous hydrogen. Thus the combination of reduction using n -butyllithium and oxidation using H 2 O leads to a complex process enlisting also a replacement of lattice oxygen by some H 2 O molecules, which enforces the expansion of the interlayer gaps. Fig. 1: Structure and composition analysis of α-MoO 3 and e-MoO 3 . a Schematic representation of expansion process from pristine α-MoO 3 (left), reaction with n -butyllithium (middle), to e-MoO 3 with H 2 O molecules located at the oxygen-defect sites (right). White: Mo; Red: O; Purple: Li; Blue: H. b Digital photos of α-MoO 3 (left) and e-MoO 3 (right). c Rietveld refinement of XRD pattern and d high-resolution TEM image for e-MoO 3 .Scale bar in d 50 nm. e Mo 3d XPS profiles of α-MoO 3 and e-MoO 3 . f TGA curves of α-MoO 3 and e-MoO 3 measured in nitrogen and air atmosphere. g Calculated increment in b -lattice parameter induced by H 2 O intercalation. The value is also compared with the calculated value of oxygen-defective MoO 3− x (Mo 16 O 47 ) and experimental value. Full size image The comparison of X-ray diffraction (XRD) patterns confirms the expansion of the interlayer space. The diffraction data of pristine α-MoO 3 (Supplementary Fig. 1 and Supplementary Note 1 ) are indexed to JCPDS card no. 05-0508. It crystallizes in the orthorhombic system (SG: Pbnm) with the refined lattice parameters of a = 3.96 (6) Å, b = 13.85 (1) Å, c = 3.70 (5) Å. e-MoO 3 maintains similar peaks of α-MoO 3 with relatively broad peak width and, more importantly, shows (0 k 0) peaks shifted toward lower angles (Fig. 1c ). These peaks refer to an enlarged b value of 15.02 (3) Å, while a and c parameters stay almost unchanged ( a = 4.08 (3) Å, c = 3.75 (2) Å). This result indicates an impressive expansion of the interlayer distance by 0.6 Å, largely higher than the 0.1 Å expansion reported for oxygen deficient α-MoO 3 compound [26] . Thus the wide interlayer distance in e-MoO 3 reported here is far above the interlayer distance solely induced by the oxygen vacancies. High-resolution transmission electron microscopic (TEM) and scanning electron microscopic (SEM) images (Fig. 1d and Supplementary Fig. 2 ) confirm that e-MoO 3 retains the nanowire structure but with a rougher surface with numerous cracks, in agreement with mechanical strains induced by the large expansion of interlayer space. To elucidate the composition evolution along with interlayer gap expansion, Fourier transform infrared (FTIR) and Raman measurements have been conducted for α-MoO 3 and e-MoO 3 (Supplementary Fig. 3 and Supplementary Note 2 ). Compared with the FTIR and Raman peaks of MoO 3 , the remarkable change observed for e-MoO 3 indicates the obvious crystal re-arrangement of the [MoO 6 ] octahedra bilayers in e-MoO 3 . Electron paramagnetic resonance (EPR) spectra of both α-MoO 3 and e-MoO 3 were measured at a low temperature of 90 K (Supplementary Fig. 4 ). In contrast to α-MoO 3 , e-MoO 3 displays an apparent signal with a g value of 1.93 and a line width of 49 Gs, which can be assigned to the presence of Mo 5+ donor levels close to the conduction band [28] , [29] . Consistent result is identified in Mo 3d X-ray photoelectron spectroscopy (XPS) data of e-MoO 3 with newly appeared Mo 5+ 3d 3/2 and 3d 5/2 peaks (234.7 and 231.5 eV, respectively, Fig. 1e ) [19] , [26] . The atomic ratio between Mo 5+ and Mo 6+ reaches approximately 3:2. Comparison of O 1s XPS spectra (Supplementary Fig. 5 ) shows the presence of an extra peak at 532.4 eV for e-MoO 3 in addition to the peak located at 530.7 eV observed in α-MoO 3 which is characteristic of lattice oxygen [30] . This confirms the presence of incorporated H 2 O in e-MoO 3 sample, and the atomic percentage of O in the incorporated H 2 O accounts for about 10% of total O atoms. No Li 1s signal is detected for e-MoO 3 , ruling out the possible pre-lithiation in e-MoO 3 (Supplementary Fig. 6 ). This is consistent with the XRD patterns of e-MoO 3 after annealing in either N 2 or air, where no Li-containing compound is observed (Supplementary Fig. 7 and Supplementary Note 3 ). Thus, based on XPS analyses, the surface composition of e-MoO 3 can be roughly estimated as MoO 2.7 ·0.3 H 2 O. Thermogravimetry analysis (TGA, Fig. 1f ) of e-MoO 3 in the air was conducted to estimate the amount of incorporated H 2 O in the whole sample. It presents the loss of intercalated water occurring at ~250 °C (mass retention of 99.12%) and the re-oxidation of oxygen-deficient MoO 3 in the temperature range of 250–460 °C (mass retention of 100.06%), which is indicative of the formula MoO 2.92 ·0.07 H 2 O for e-MoO 3 . From both XPS and TGA analysis, we notice that the molar amount of oxygen defects is approximately equal to that of the incorporated H 2 O molecules. Thus we consider that the incorporated H 2 O molecules take the place of lattice O of e-MoO 3 , functioning as buffered spacer to stabilize the widened interlayer gaps between the layers. This assumption is further supported by the density functional theory (DFT) simulation, which is performed employing the bulk supercells of Mo 16 O 48− x · x H 2 O ( x = 1–6, which represents the number of the incorporated H 2 O molecules) shown in Supplementary Figs. 8 and 9 . Notably, an increment of 0.9 Å in the b -lattice parameter is revealed even when one lattice O is replaced by one H 2 O molecule (Fig. 1g ). By contrast, for the sample with only oxygen defects (Mo 16 O 47 ), the increment can only reach 0.13 Å, which further confirms the dominant role of the incorporated H 2 O in expanding the interlayer gaps. When x is between 3 and 6 (corresponding to MoO 2.81 ·0.19 H 2 O to MoO 2.63 ·0.37 H 2 O), the calculated increment in the b -lattice parameter agrees well with our experimental XRD results. In addition, the simulated e-MoO 3 structure with most stable configuration also reveals that the incorporated H 2 O induces the distortion of the [MoO 6 ] octahedra (Supplementary Fig. 10 ), leading to substantial changes in O–O distances (both intra- and inter-layer ones, Supplementary Fig. 11 and Supplementary Note 4 ). The increment in band density near the Fermi level for e-MoO 3 compared with α-MoO 3 is evidenced by the ultraviolet photoelectron spectroscopy analysis (Supplementary Figs. 12 and 13 and Supplementary Note 5 ) and O K -edge X-ray absorption near-edge structure spectra (Supplementary Fig. 14 and Supplementary Note 6 ). e-MoO 3 sample exhibits a remarkable conductivity of 0.95 S m −1 at 300 K as determined by the van der Pauw 4-probe method (Supplementary Fig. 15 ), whereas the conductivity of pristine α-MoO 3 was too low to be detected. The enhanced conductivity can be explained by the narrowed band gap and the increment in the carrier concentration (Supplementary Fig. 16 and Supplementary Note 7 ), which can be attributed to the electron hopping mechanism boosted by Mo 5+ [31] , [32] . Enhanced Li + storage kinetics of e-MoO 3 e-MoO 3 sample with large opened interlayer space has been used as electrode material for Li-ion intercalation reaction. 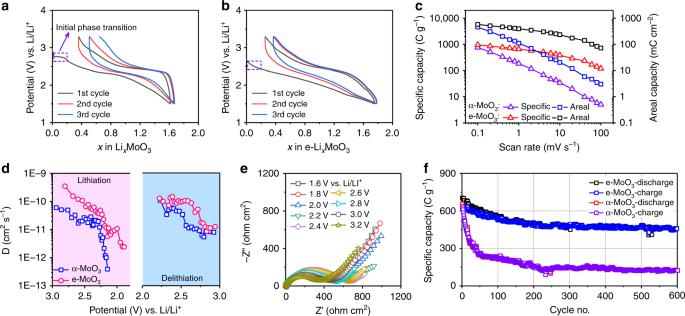Fig. 2: Li+storage behavior of α-MoO3and e-MoO3electrodes. Initial three galvanostatic charge/discharge profiles ofaα-MoO3andbe-MoO3electrodes.cSpecific and areal capacity as a function of scan rate.dLi+diffusion coefficient calculated from GITT curves.eNyquist plots of e-MoO3at different potentials.fCycling performance of α-MoO3and e-MoO3at 100 mA g−1. Figure 2a, b compares the initial three galvanostatic charge/discharge cycles at 50 mA g −1 in 2 M LiPF 6 dissolved in ethyl methyl carbonate electrolyte. The first lithiation process of α-MoO 3 starts with a short constant potential plateau at about 2.75 V vs. Li/Li + , which is consistent with the presence of a reduction peak in the first cathodic cyclic voltammetry (CV) cycle (Supplementary Fig. 17 ). This process is related to an irreversible phase transition and will be later discussed in more detail in the in operando XRD section. By contrast, such a feature is not observed in the first lithiation reaction of e-MoO 3 , identifying the role of the widened interlayer gaps in inhibiting the phase transition. Also, the Coulombic efficiency of e-MoO 3 in the first cycle (85%) is found to be higher than that of α-MoO 3 (78%). Such an improvement is also observed during the next cycles (Fig. 2a, b ). Fig. 2: Li + storage behavior of α-MoO 3 and e-MoO 3 electrodes. Initial three galvanostatic charge/discharge profiles of a α-MoO 3 and b e-MoO 3 electrodes. c Specific and areal capacity as a function of scan rate. d Li + diffusion coefficient calculated from GITT curves. e Nyquist plots of e-MoO 3 at different potentials. f Cycling performance of α-MoO 3 and e-MoO 3 at 100 mA g −1 . Full size image CV curves from a scan rate range of 0.1–100 mV s −1 were collected for both α-MoO 3 and e-MoO 3 electrodes with similar weight loadings (Supplementary Fig. 18 ). As revealed in Fig. 2c , e-MoO 3 depicts both higher capacity and better rate capability than α-MoO 3 . At an extremely slow scan rate of 0.1 mV s −1 , the capacity of e-MoO 3 electrode is close to the theoretical capacity (1005 C g −1 , 279 mAh g −1 ), while α-MoO 3 electrode only shows a capacity of 756 C g −1 (210 mAh g −1 ). Importantly, our e-MoO 3 electrode delivers an outstanding areal capacity of 578 mC cm −2 , drastically outperforming the reported state-of-the-art α-MoO 3 -based pseudocapacitive electrodes [19] , [22] , [25] , [26] , [33] . When the scan rate increases to 10 and 100 mV s −1 , e-MoO 3 can maintain high capacities of 233 and 72 mC cm −2 , respectively, indicating high power capability. As for α-MoO 3 electrode, the capacity at 10 and 100 mV s −1 can only reach 20 and 3 mC cm −2 , respectively. Moreover, galvanostatic charge/discharge profiles at different rates also verify the superior rate capability of e-MoO 3 electrode (Supplementary Fig. 19 ). The significant role of the incorporated H 2 O molecules in accelerating the diffusion of Li + within e-MoO 3 lattice was further studied. Figure 2d compares the Li + diffusion coefficient ( D ) of α-MoO 3 and e-MoO 3 obtained by employing a galvanostatic intermittent titration technique (GITT, see Supplementary Figs. 20 and 21 ). The D Li+ values in e-MoO 3 electrode (2.4 × 10 −12 –3.5 × 10 −10 cm 2 s −1 ) are substantially higher than those in α-MoO 3 electrode (3.9 × 10 −13 –6.0 × 10 −11 cm 2 s −1 ). The fastened Li + diffusion can be assigned to both the expanded ionic diffusion channels and the shielding effect of incorporated H 2 O that screens the electrostatic interaction between Li + and MoO 3 lattice [34] , [35] . Meanwhile, we measured the electrochemical impedance spectroscopy for both α-MoO 3 (Supplementary Fig. 22 ) and e-MoO 3 (Fig. 2e ) at various potentials from the cathodic process. Both electrodes depict stable ohmic resistance ( R s ) and V-shape variation for charge transfer resistance ( R ct ) along with the change of potential (Supplementary Fig. 23 ). It can be observed that R s , R ct , and the overall resistance of e-MoO 3 are all lower than those of α-MoO 3 , further justifying the improved charge and ion transfer efficiency for e-MoO 3 . In addition, e-MoO 3 electrode exhibits a significant improvement in cycling stability compared to α-MoO 3 (Fig. 2f ). When cycled at 100 mA g −1 for 600 cycles, e-MoO 3 still maintains a high capacity of 455 C g −1 , delivering excellent capacity retention of 71%. In contrast, α-MoO 3 electrode shows rapid capacity decay, from 586 C g −1 in the first cycle to 175 C g −1 after only 50 cycles. To gain insight into the performance superiority of e-MoO 3 to pristine α-MoO 3 , we further carried out in operando XRD characterizations of electrodes during the first three lithiation/de-lithiation cycles. During the initial lithiation (Fig. 3a ), α-MoO 3 electrode experienced an irreversible phase transition at 2.75 V vs. Li/Li + , which was evidenced by the rapid disappearance of the (0 k 1 0) peaks of the pristine α-MoO 3 and the appearance of a set of broad (0 k 2 0) peaks belonging to the lithiated MoO 3 (Li x MoO 3 ). This irreversible phase transition results in a sudden distortion of the layers in α-MoO 3 , which accounts for the fast structural collapse and sluggish kinetics of α-MoO 3 [36] . Although limited information can be gained for e-MoO 3 from XRD peaks within 15–35° due to the overlap of multiple peaks, one can clearly notice that the primitive (020) and (060) peaks of e-MoO 3 were well maintained during the whole lithiation/de-lithiation process (Fig. 3b ). This result suggests a stable structural phase resulting from the expanded interlayer gaps in e-MoO 3 . We further compare the shift of the (0 k 0) peak of α-MoO 3 and e-MoO 3 located between 10° and 14° during the second and third lithiation/de-lithiation cycles (Fig. 3c, d ), which is directly associated with the volume change of the lattice in b direction. Benefiting from the lessened electrostatic interaction between Li + and MoO 3 lattice, the peak shift of e-MoO 3 (0.8°) during the second cycle is apparently smaller than that of α-MoO 3 (1.3°). Besides, almost no difference is observed between the peaks of e-MoO 3 at the beginning of the second cycle and at the end of the third cycle, while α-MoO 3 displays a peak shift of 0.6°. Thus we conclude that the incorporated H 2 O molecules efficiently alleviate the volume change of e-MoO 3 and prevent the structure collapse during Li + insertion/extraction, which also explains the enhanced cycling performance of e-MoO 3 with respect to α-MoO 3. Moreover, aside from α-MoO 3 , we also demonstrated the feasibility of our H 2 O-incorporation strategy in improving the charge storage ability of birnessite δ-MnO 2 for Zn-ion aqueous batteries (Supplementary Figs. 24 and 25 and Supplementary Note 8 ). 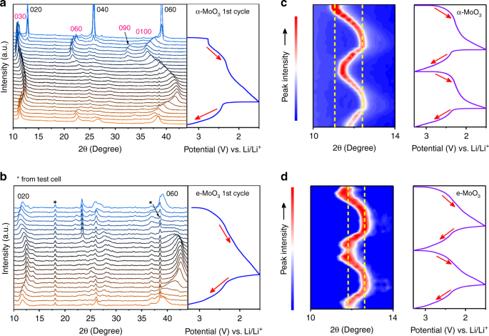Fig. 3: In operando XRD study. In operando XRD measurements ofa,cα-MoO3andb,de-MoO3electrodes duringa,bthe first galvanostatic lithiation/de-lithiation cycle andc,dthe second and third cycles. Fig. 3: In operando XRD study. In operando XRD measurements of a , c α-MoO 3 and b , d e-MoO 3 electrodes during a , b the first galvanostatic lithiation/de-lithiation cycle and c , d the second and third cycles. Full size image Full DIES device Full DIES device was further assembled by e-MoO 3 anode, graphite cathode and 2 M LiPF 6 in ethyl methyl carbonate electrolyte to demonstrate the practical application of our e-MoO 3 electrode in constructing full device. As anion-intercalation graphite cathode owns a high anion-intercalation potential (average discharge potential: 4.6 V), a large specific capacity (396 C g −1 at 50 mA g −1 ), and importantly high charge-storage kinetics (almost no capacity decay from 50 to 500 mA g −1 , Supplementary Fig. 26 and Supplementary Note 9 ), the designed e-MoO 3 //graphite device holds the opportunity to mitigate the inherent trade-off between energy density and power density for energy storage devices. According to the specific capacity of e-MoO 3 anode and graphite cathode at a low rate, a cathode/anode mass ratio of 2.5 was used to assemble the dual-ion-intercalation device (Fig. 4a ), and a theoretical capacity of 275 C g −1 is expected for the cell based on the total mass of active materials. From the experiments, a reversible capacity of 200 C g −1 (72.7% of theoretical capacity) could be achieved at 100 mA g −1 (based on the mass of e-MoO 3 ) within a 1.0–3.5 V voltage range. Fig. 4: e-MoO 3 //graphite DIES device. a Design of the dual-ion-intercalation MoO 3 //graphite cell. On the anode side, predominantly Li + is intercalated and de-intercalated between [MoO 6 ] layers of MoO 3 during charge/discharge. On the cathode side, graphite is used as a host for hexafluorophosphate (PF 6 − ) anion intercalation/de-intercalation. b The initial four galvanostatic charge/discharge cycles at 100 mA g −1 and the corresponding potential variation of the cathode and anode. c CV curves of the device at different scan rates. d Change of the gravimetric capacity based on the total active mass as a function of v −1/2 . e Rate performance of the e-MoO 3 //graphite device based on the volume of the whole device. f Ragone plots of e-MoO 3 //graphite device in comparison with state-of-the-art electrochemical energy storage devices; the performance is normalized to the total cell volume, which includes the active materials, current collectors and separators. g Cycling performance of the e-MoO 3 //graphite device at 400 mA g −1 and 1 A g −1 . 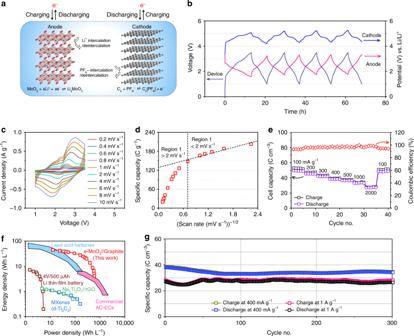Fig. 4: e-MoO3//graphite DIES device. aDesign of the dual-ion-intercalation MoO3//graphite cell. On the anode side, predominantly Li+is intercalated and de-intercalated between [MoO6] layers of MoO3during charge/discharge. On the cathode side, graphite is used as a host for hexafluorophosphate (PF6−) anion intercalation/de-intercalation.bThe initial four galvanostatic charge/discharge cycles at 100 mA g−1and the corresponding potential variation of the cathode and anode.cCV curves of the device at different scan rates.dChange of the gravimetric capacity based on the total active mass as a function ofv−1/2.eRate performance of the e-MoO3//graphite device based on the volume of the whole device.fRagone plots of e-MoO3//graphite device in comparison with state-of-the-art electrochemical energy storage devices; the performance is normalized to the total cell volume, which includes the active materials, current collectors and separators.gCycling performance of the e-MoO3//graphite device at 400 mA g−1and 1 A g−1. Full size image Figure 4b shows the first four galvanostatic charge/discharge cycles using a Li metal reference electrode to record the anode and cathode potentials during the cell cycling. After the first two cycles, the potential windows for anode and cathode stabilize as 1.8–3.3 and 4.3–5.3 V vs. Li/Li + , respectively (Fig. 4b ). At the end of charge and discharge, the cathode and anode are close to its upper potential limit (3.3 V vs. Li/Li + for e-MoO 3 , 5.3 V vs. Li/Li + for graphite), respectively. The unexploited capacity (capacity at a potential <1.8 V for e-MoO 3 and <4.3 V for graphite) explains the lower capacity of the device compared with the theoretical values. Noteworthy is that the Coulombic efficiency of e-MoO 3 anode (85%) at the first cycle is close to that of graphite cathode (75%, Supplementary Fig. 27 ), so that the two electrodes in the full cell provide suitable buffers for each other during the initial polarization. Moreover, the anode potential is far above the Li plating potential, which can effectively prevent the safety issue associated with metal dendrite growth. CV curves recorded from 0.2 to 100 mV s −1 (discharge time from 3.5 h to 25 s) present multi-pairs of redox peaks, corresponding to different steps of anion and cation intercalation/de-intercalation (Fig. 4c and Supplementary Fig. 28 ). To establish the rate-limiting step of the charge storage process, Fig. 4d plots the specific capacity based on the total active mass as a function of v −1/2 [37] . At a low scan rate of 0.2 mV s −1 , the capacity is up to 222 C g −1 . Along with the increasing scan rate, there are two distinct regions. At scan rates <2 mV s −1 , the charge storage is almost not limited by the solid-state ion diffusion, thus the capacity is mostly independent on the scan rate. The extrapolated y -intercept capacity, that is, the charge storage from capacitive processes at the infinite scan rate, reaches around 130 C g −1 . The high kinetics of the device is also reflected by the slope of the plots of log ( i ) vs. log ( v ) for the main redox peaks (Supplementary Fig. 29 and Supplementary Note 10 ). We further studied the rate performance of the DIES device from 100 mA g −1 to 2 A g −1 (Fig. 4e ). The capacity based on the total cell stack volume (illustrated in Supplementary Fig. 30 and Supplementary Note 11 ) reaches 49 C cm −3 (200 C g −1 , Supplementary Fig. 31 ) at 100 mA g −1 , and 55% capacity was maintained when the current density increased to 2 A g −1 (a discharge time of 3.2 min). The Ragone plot shown in Fig. 4f compares the volumetric performance of the cell with the state of the art of electrochemical energy storage devices (Supplementary Fig. 32 shows the performance normalized to the active material weight). The present e-MoO 3 //graphite device could deliver an energy density up to 44 Wh L −1 , which outperforms those of Li thin-film micro-battery [38] , Na-ion capacitors [39] , activated carbon- [40] and MXene-based [41] supercapacitors, and is comparable to those of lead-acid batteries [42] . Meanwhile, a decent maximum power density of 600 W L −1 was achieved, close to supercapacitor-level power densities. Finally, cycling stability was evaluated by galvanostatic charge/discharge tests (Fig. 4g ). Impressive cycling stability with 90% and 97% capacity retention was observed over 300 cycles at 400 and 1000 mA g −1 . Note that both the volumetric and gravimetric capacities of graphite are substantially lower than those of e-MoO 3 , which consequently limit the energy storage capability of the whole DIES device. Li-ion full cell was also assembled by e-MoO 3 anode and commercial LiCoO 2 cathode (Supplementary Fig. 33 and Supplementary Note 12 ). Although the maximum energy density of e-MoO 3 //LiCoO 2 device (146 Wh kg −1 ) is slightly higher than that of e-MoO 3 //graphite device (133 Wh kg −1 ), the power density of e-MoO 3 //LiCoO 2 is far below that of e-MoO 3 //graphite device. As a result, developing a new cation-intercalation cathode with comparable specific capacity with e-MoO 3 anode would be beneficial for further boosting the energy and power densities of full devices. In summary, we demonstrated an efficient H 2 O-incorporation strategy for expanding the interlayer gaps of α-MoO 3 , which triggers a robust Li + storage ability with significantly improved rate capability and prolonged cycling stability. There are three key advantages of our strategy. First, the incorporated H 2 O molecules function as effective spacers to stabilize the expanded interlayer gaps in e-MoO 3 , which provides efficient Li + diffusion channels and avoid the irreversible phase transition of e-MoO 3 during the initial lithiation process. Second, the H 2 O molecules can shield electrostatic interaction between Li + and e-MoO 3 lattice, thus alleviating the volume change of e-MoO 3 during repeated Li intercalation/de-intercalation and improving the cycling stability of e-MoO 3 . Third, since the incorporated H 2 O molecules take the place of lattice O and the molecular mass of H 2 O is very close to O, the improved rate capability and cycling stability of e-MoO 3 come without the sacrifice of specific capacity. Moreover, a DIES device was assembled by coupling cation-intercalation e-MoO 3 and anion-intercalation graphite. Such a device links the intercalation-type charge storage with fast kinetics, which thus can bring together high power density (up to 600 W L −1 ) and energy density (up to 44 Wh L −1 ). This study offers insightful understanding of the interlayer gap-engineering strategy to improve the ion-intercalation chemistry of layered electrode materials, which opens opportunities for the next-generation energy storage technologies. Materials All chemicals were of analytical grade and used directly without any purification. Ammonium molybdate tetrahydrate ((NH 4 ) 6 Mo 7 O 24 ·4H 2 O), lithium cobalt oxide (LiCoO 2 ), concentrated HNO 3 (70 wt%), n-butyl lithium in hexane, hexane, Li foil, graphite flakes (average size 20 µm), sodium alginate, Super P carbon black, and 2 M LiPF 6 in ethyl methyl carbonate were purchased from Sigma-Aldrich. Material preparation α-MoO 3 nanowires were prepared through a hydrothermal method. In all, 6.5 g of (NH 4 ) 6 Mo 7 O 24 ·4H 2 O was first dissolved into 180 mL of distilled water. Then 30 mL concentrated HNO 3 (70 wt%) was added into the solution, followed by vigorous stirring. The obtained solution was then transferred into a 250-mL Teflon-lined stainless autoclave and heated in an electric oven at 180 °C for 12 h. After naturally cooled down to room temperature, the obtained powder sample was washed thoroughly with distilled water and dried in a vacuum oven at 80 °C for 12 h. e-MoO 3 was obtained by dispersing 500 mg of α-MoO 3 nanowires in 16 mL of 0.8 M n-butyl lithium in hexane. The mixture was then stirred for 24 h at room temperature under the protection of inert argon atmosphere. The lithiated compound was separated by vacuum filtration and washed several times with hexane. Subsequently, the sample was placed in 100 mL of distilled water and stirred for half an hour. Finally, the sample was centrifuged and dried in a vacuum oven at 80 °C for 12 h. Electrochemical measurements All the half-cell tests were conducted in CR2032 coin-type cells. To prepare the electrodes, active materials (α-MoO 3 , e-MoO 3 , and graphite), binder (sodium alginate), and Super P carbon black were mixed with a weight ratio of 8:1:1. The mixture was dispersed in water and coated on a Cu foil (α-MoO 3 , e-MoO 3 ) or an Al foil (graphite), followed by drying at 80 °C for 12 h under vacuum. The loading mass of α-MoO 3 and e-MoO 3 is about 0.6 ± 0.1 mg cm −2 , while the loading mass of graphite is 1.5 ± 0.1 mg cm −2 . The coin cells were assembled using Li metal foil as a counter electrode, Celgard 2400 as the separator, and 2 M LiPF 6 dissolved in ethyl methyl carbonate as the electrolyte. The full-cell tests were performed with a three-electrode stainless steel Swagelok cell. e-MoO 3 coated on Cu foil and graphite coated on Al foil were used as anode and cathode, respectively, with a mass ratio of 1:2.5. A Li metal foil was inserted as a reference electrode to monitor the potential variation of both anode and cathode. All cell assembly was carried out in an argon-filled glove box, and the concentration of O 2 and H 2 O were kept <0.1 ppm. The charge–discharge curves were collected from a Land battery test system (LAND CT2001A) at room temperature. GITT test was performed with a galvanostatic charge/discharge pulse of 50 mA g −1 for 10 min, followed by an open circuit step for 3 h. Both CV and electrochemical impedance measurements were conducted on a VMP3 potentiostat (Biologic, USA). The electrochemical impedance measurements were carried out at a 10 mV ac oscillation amplitude over the frequency range of 100 kHz to 0.01 Hz. Characterization The microstructures and compositions of samples were analyzed by field-emission SEM (Carl Zeiss Gemini 500), TEM (FEI Tecnai G 2 F30), XRD (Bruker D8) using Cu Kα radiation ( λ = 0.154 nm), and TGA (Netzsch DSC-204 F1). Raman spectra were measured on a NTMDT confocal spectrometer with a 532-nm laser, and the spot size of the laser beam was ~0.5 μm. Infrared spectra were recorded on a FT-IR Spectrometer Tensor II (Bruker) with an ATR unit. EPR measurement was performed in the X -band (9.32 GHz) with 1.0 G modulation amplitude and a magnetic field modulation of 100 kHz using a Bruker, A300-10-12 Bruker EPR spectrometer at 90 K. XPS, near-edge X-ray absorption fine structure (NEXAFS), and ultraviolet photoemission spectroscopy were measured at the Photoemission Endstation (BL10B beamline) of the National Synchrotron Radiation Laboratory (NSRL) in Hefei, China. Briefly, the beamline is connected to a bending magnet and equipped with three gratings that cover photon energies from 100 to 1000 eV with a typical photon flux of 1 × 10 10 photons/s and a resolution ( E / ΔE ) better than 1000 at 244 eV. XPS spectra were collected using monochromatic Mg-Kα X-ray (1254.6 eV) as the excitation source. NEXAFS spectra were recorded in the total electron yield mode using a sample current measurement. To detect the conductivity, 10 mg sample was first dispersed in ethanol and coated on a cellulose membrane (diameter of 4.5 cm) through vacuum filtration. The membrane loaded with sample was cut into a size of 1 × 1 cm 2 , and then a four-point contact was placed on the surface to define a square. The I – V curves were measured in van der Pauw geometry under vacuum at varied temperatures (from 100–400 K) using a commercial Lakeshore Hall System. A two-electrode Swagelok cell was used for in operando XRD tests. Freestanding α-MoO 3 or e-MoO 3 film consisting of 90 wt% of active material, 5 wt% of Super P, and 5 wt% of polytetrafluoroethylene was placed onto a beryllium foil acting as the current collector, and a Li foil was used as the counter electrode. XRD test was carried out on a Bruker D8 advance diffractometer in the 10–50° 2 θ range with a step of 0.0152°, while the electrode was undergoing a galvanostatic charge/discharge test at 50 mA g −1 . Computational details All calculations were performed using the plane-wave DFT code available in the Vienna Ab initio Simulation Package (VASP) within the generalized gradient approximation, using the Perdew–Burke–Ernzerhof functional for the exchange and correlation potential. Spin polarized calculations were performed to account for orbit coupling. The electronic wave functions were described in the projected augmented wave formalism, and a real-space projection was further used for the total wavefunction analysis. The cutoff energy for plane-wave basis set was set to 400 eV. All atomic positions and lattice vectors were fully optimized using a conjugate gradient algorithm to obtain the unstrained configuration. Atomic relaxation was performed until the change of total energy was <1 × 10 −5 eV, and all the forces on each atom were <0.01 eV Å −1 . The orthorhombic cell with space group Pbnm was used for α-MoO 3 . Supercells containing 2 × 1 × 2 conventional cells (16 formula units, Supplementary Figs. 7 and 8 ) were used to calculate energies and band structure, in which Monkhorst–Pack scheme k -point grid was set to 5 × 3 × 5.